Temporal identity transition from Purkinje cell progenitors to GABAergic interneuron progenitors in the cerebellum In the cerebellum, all GABAergic neurons are generated from the Ptf1a-expressing ventricular zone (Ptf1a domain). However, the machinery to produce different types of GABAergic neurons remains elusive. Here we show temporal regulation of distinct GABAergic neuron progenitors in the cerebellum. Within the Ptf1a domain at early stages, we find two subpopulations; dorsally and ventrally located progenitors that express Olig2 and Gsx1, respectively. Lineage tracing reveals the former are exclusively Purkinje cell progenitors (PCPs) and the latter Pax2-positive interneuron progenitors (PIPs). As development proceeds, PCPs gradually become PIPs starting from ventral to dorsal. In gain- and loss-of-function mutants for Gsx1 and Olig1/2 , we observe abnormal transitioning from PCPs to PIPs at inappropriate developmental stages. Our findings suggest that the temporal identity transition of cerebellar GABAergic neuron progenitors from PCPs to PIPs is negatively regulated by Olig2 and positively by Gsx1, and contributes to understanding temporal control of neuronal progenitor identities. The cerebellum represents a good model system to investigate the molecular machinery underlying specification of neuron subtypes, because it comprises several neuronal types that are distinct in terms of their morphological, physiological and immunohistochemical features. During development, the neuroepithelium of the alar plate of rhombomere 1 generates all cerebellar neuron types [1] , [2] , [3] , [4] . Cerebellar neuron-producing neuroepithelium can be divided into two regions; the rhombic lip and the ventricular zone (VZ). All types of cerebellar GABAergic neurons are generated from the VZ that expresses the basic helix-loop-helix (bHLH) transcription factor, pancreatic transcription factor 1a (Ptf1a) that is required for GABAergic neuron production [5] . Coincidently, Machold et al. [6] and Wang et al. [7] reported that cerebellar glutamatergic neurons are derived from the rhombic lip that expresses Atoh1, which is indispensable for producing glutamatergic neurons. Among cerebellar GABAergic neurons, there are several types of neurons that have distinct characteristics. While Purkinje cells are projection neurons that express Corl2/Skor2 from early developmental stages [8] , all cerebellar interneurons (INs) such as Golgi, stellate, basket cells and INs in the deep cerebellar nuclei (DCN) express Pax2 (ref. 9) [9] . Therefore, we will refer to cerebellar GABAergic interneurons as ‘Pax2+ INs’ in this report. The mechanisms that specify each GABAergic subtype remains unclear. Birthdating studies using 3 H-thymidine and BrdU [10] , [11] , [12] , [13] , [14] , [15] , as well as adenovirus [16] have revealed that each type of neuron is generated at distinct developmental stages. Purkinje cells appear relatively early (E10.5~13.5 in mice), Golgi cells a little later (E13.5~postonatal day 0) and stellate/basket cells mainly perinatally. In addition, somatic recombination-based clonal analyses suggested that Purkinje, Golgi and basket/stellate cells belong to the same lineage [17] , [18] . These data indicate that some temporal information in the Ptf1a-expressing neuroepithelial domain (Ptf1a domain) may be involved in specification of neuronal types. However, the underlying molecular mechanisms have yet to be defined. Heterochronic transplantation studies have also provided important clues to understanding cerebellar development [19] . It has been shown that tissues or dissociated cells taken from cerebellar primordium at early neurogenesis stages can differentiate into all types of cerebellar GABAergic neurons, while those from postnatal cerebellum differentiated only into GABAergic Pax2+ INs [20] , [21] . These findings suggested that, while cerebellar primordium at early stages may contain GABAergic neuron progenitors that can give rise to all types of cerebellar GABAergic neurons including Purkinje cells and Pax2+ INs, cerebellar anlage at later stages contain GABAergic neuron progenitors that produce only Pax2+ INs. Although these observations imply that different types of cerebellar GABAergic progenitors have distinct temporal identities, the molecular machinery involved in regulating temporal information remains unclear. The homeodomain-containing transcription factor, Gsx1/Gsh1, is known to be expressed in some brain regions including telencephalon and diencephalon [22] . Although targeted disruption of the Gsx1 gene causes pleiotropic abnormalities in pituitary development and results in dwarfism and sexual infantilism [23] , its function in other brain regions is not well defined. The bHLH transcription factor, Olig2, was first identified as an oligodendrocyte-specific transcription factor and later as an essential factor for specification of motor neurons derived from the pMN domain of the spinal cord [24] , [25] , [26] , [27] . Although Olig2 is also expressed in the VZ of cerebellum [28] , its function there is unclear. In this study, we identify two distinct populations of GABAergic neuron progenitors in the Ptf1a domain; dorsally and ventrally located progenitors that express Olig2 and Gsx1, respectively. The former are exclusively Purkinje cell progenitors (PCPs) and the latter Pax2+ IN progenitors (PIPs). As development proceeds, PCPs gradually become PIPs starting from ventral to dorsal. Results from loss-of- as well as gain-of-function experiments suggest the roles for Olig2 and Gsx1 in the regulation of the temporal identity transition of GABAergic neuron progenitors from PCPs to PIPs during cerebellar development. Expression of Olig2 and Gsx1 in the Ptf1a domain Previously, Chizhikov et al. [29] defined four cellular populations (denoted c1–c4 domains) in the cerebellar primordium via the expression of a few transcription factors. They showed that all cerebellar GABAergic neurons express transcription factors Lhx1 and Lhx5 (Lhx1/5), which constitute the c2 domain located just above the Ptf1a domain, which is consistent with the finding that all cerebellar GABAergic neurons emerge from the Ptf1a domain [5] . Furthermore, at the early neurogenesis stages (for example, embryonic day (E) 12.5 in mice), we previously subdivided the c2 domain into dorsally (c2d) and ventrally (c2v) located subdomains that express Corl2 and Pax2, respectively [8] . This raised the possibility that Purkinje cells and Pax2+ INs are produced from distinct progenitor regions within the Ptf1a domain. Therefore, we looked for transcription factors that are expressed differentially along the dorsoventral axis within the Ptf1a domain. We found that Gsx1 and Olig2 are exclusively expressed in cells of the ventral and dorsal parts of the Ptf1a domain at E12.5, respectively ( Fig. 1a–d ). Even in the boundary region, we could not detect any cells that expressed both transcription factors simultaneously ( Fig. 1e–g ). 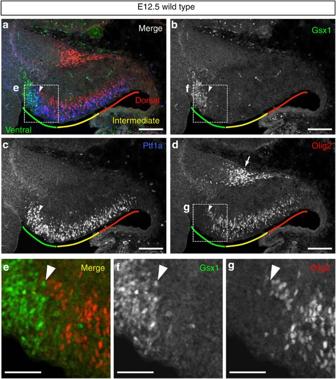Figure 1: Mutually exclusive expression of Olig2 and Gsx1 in the cerebellar VZ at E12.5. (a–d) Wild-type cerebellar primordium at E12.5 stained with antibodies for Gsx1, Olig2 and Ptf1a. Coloured lines indicate ventral (green), intermediate (yellow) and dorsal (red) regions of cerebellar VZ, respectively. Arrowheads indicate the boundary between Gsx1 and Olig2-expressing progenitors. (e–g) Higher-magnification images of the rectangular regions in (a), (b) and (d), respectively. Scale bars represent (a–d) 100 μm, (e–g) 50 μm. Figure 1: Mutually exclusive expression of Olig2 and Gsx1 in the cerebellar VZ at E12.5. ( a – d ) Wild-type cerebellar primordium at E12.5 stained with antibodies for Gsx1, Olig2 and Ptf1a. Coloured lines indicate ventral (green), intermediate (yellow) and dorsal (red) regions of cerebellar VZ, respectively. Arrowheads indicate the boundary between Gsx1 and Olig2-expressing progenitors. ( e – g ) Higher-magnification images of the rectangular regions in ( a ), ( b ) and ( d ), respectively. Scale bars represent ( a – d ) 100 μm, ( e – g ) 50 μm. Full size image Progenitors for Purkinje cells and Pax2+ INs At E12.5, the Olig2+ region is much larger than that with Gsx1+ cells ( Fig. 1a–d ). Olig2 expression was also observed in the pial side of the cerebellum (arrow in Fig. 1d ), but that will not be discussed here. At E12.5, Purkinje cells were found just above the Olig2+ cells ( Supplementary Fig. 1a ), while Pax2+ INs were localized above the Gsx1+ cells ( Supplementary Fig. 1b ). These findings suggest that Purkinje cells and Pax2+ INs arise from the Olig2+ and Gsx1+ cells in the Ptf1a domain. Next, we performed short-term lineage trace analyses using Olig2 GFP/+ and Gsx1 GFP/+ mice ( Supplementary Fig. 2 ). Because the half-life of GFP is relatively longer than the transcription factors [30] , we can label cells derived from Olig2+ and Gsx1+ cells using GFP expressed under the control of endogenous Olig2 and Gsx1 promoters, respectively. In the E12.5 cerebella of Olig2 GFP/+ embryos, GFP-labelled cells derived from the Olig2+ cells expressed Corl2 but not Pax2 ( Fig. 2a–d,i–l ). This indicates the Olig2+ cells are PCPs but not PIPs. In contrast, in the E12.5 cerebella of Gsx1 GFP/+ embryos, GFP-labelled cells were immunoreactive to Pax2 but not Corl2, indicating that the Gsx1+ cells are PIPs ( Fig. 2e–h,m–p ). These findings indicate that there are two kinds of GABAergic neuron progenitors within the Ptf1a domain of the cerebellar primordia: Olig2+ PCPs and Gsx1+ PIPs. 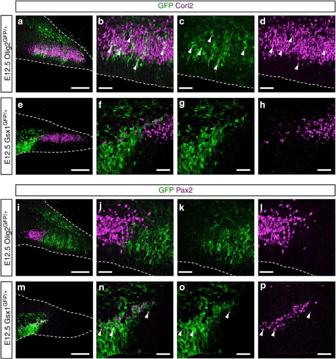Figure 2: Cerebellar progenitors for Purkinje cells and Pax2+ INs. (a–p) Lineage tracing analyses usingOlig2GFP/+(a–d,i–l) andGsx1GFP/+(e–h,m–p) embryos. (a–h) In the cerebellum, Purkinje cells are specifically labelled with an antibody for Corl2. (i–p) GABAergic interneurons are labelled with an antibody for Pax2. Arrowheads highlight double-stained cells. Stages, genotypes and antibodies are indicated. Scale bars represent (a,e,iandm) 100 μm, (b–d,f–h,j–landn–p) 25 μm. Figure 2: Cerebellar progenitors for Purkinje cells and Pax2+ INs. ( a – p ) Lineage tracing analyses using Olig2 GFP/+ ( a – d , i – l ) and Gsx1 GFP/+ ( e – h , m – p ) embryos. ( a – h ) In the cerebellum, Purkinje cells are specifically labelled with an antibody for Corl2. ( i – p ) GABAergic interneurons are labelled with an antibody for Pax2. Arrowheads highlight double-stained cells. Stages, genotypes and antibodies are indicated. Scale bars represent ( a , e , i and m ) 100 μm, ( b – d , f – h , j – l and n – p ) 25 μm. Full size image Next, we examined the dynamic change of the distribution patterns of Olig2+ and Gsx1+ progenitors at different developmental stages. As development proceeds, the region with Olig2+ progenitors gradually diminishes and disappears by E14.5. Conversely, the region with Gsx1+ progenitors expands to cover the entire Ptf1a domain by E14.5 ( Fig. 3a–d ). Coincidently, we observed that Pax2+ INs reside only in the ventral side of the cerebellum at earlier stages, and their localization expands towards the dorsal side of the cerebellum as development proceeds ( Supplementary Fig. 3a–c ). This also supports previous findings that Purkinje cells are produced until E13.5 but not at later stages [16] , [31] , [32] . To further examine the expression dynamics across the cerebellum, multiple coronal sections along the anteroposterior axis at different developmental stages were immunostained with Olig2 and Gsx1 together with Ptf1a ( Supplementary Fig. 3d ). Although the proportion of Olig2- and Gsx1-expressing areas differ along the anteroposterior axis, the regions with Olig2+ progenitors were gradually superseded by those with Gsx1+ progenitors throughout the cerebellum during development. 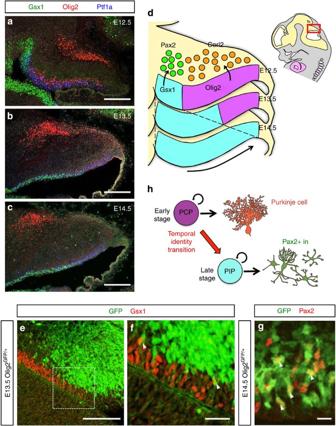Figure 3: Temporal identity transition of cerebellar GABAergic neuron progenitors. (a–d) Developmental changes of localization of PCPs and PIPs in the embryonic cerebellar VZ. (a–c) Immunostaining with Gsx1, Olig2 and Ptf1a in (a) E12.5, (b) E13.5 and (c) E14.5 cerebella. (d) Schematic diagram of developmental changes of Gsx1- and Olig2-expressing regions in the cerebellar VZ. As development proceeds, Gsx1-expressing region expands to the dorsal region, while Olig2-expressing region shrinks. (e–g) Intermediate-term lineage trace usingOlig2GFP/+embryos to investigate the lineage relationship between PCPs and PIPs. Cerebellar primordium ofOlig2GFP/+at E13.5 (e,f) or E14.5 (g) was immunostained with indicated antibodies. Arrowheads highlight double-positive cells for GFP and the marker. (f) High magnification of the rectangle in (e). (h) Schematic diagram of temporal identity transition of cerebellar GABAergic neuron progenitors from PCPs to PIPs. PCPs at early stages change their character to become PIPs at late embryonic stages and start to generate Pax2+ INs. Scale bars represent: (a–c,e) 100 μm, (f) 25 μm, (g) 10 μm. Figure 3: Temporal identity transition of cerebellar GABAergic neuron progenitors. ( a – d ) Developmental changes of localization of PCPs and PIPs in the embryonic cerebellar VZ. ( a – c ) Immunostaining with Gsx1, Olig2 and Ptf1a in ( a ) E12.5, ( b ) E13.5 and ( c ) E14.5 cerebella. ( d ) Schematic diagram of developmental changes of Gsx1- and Olig2-expressing regions in the cerebellar VZ. As development proceeds, Gsx1-expressing region expands to the dorsal region, while Olig2-expressing region shrinks. ( e – g ) Intermediate-term lineage trace using Olig2 GFP/+ embryos to investigate the lineage relationship between PCPs and PIPs. Cerebellar primordium of Olig2 GFP/+ at E13.5 ( e , f ) or E14.5 ( g ) was immunostained with indicated antibodies. Arrowheads highlight double-positive cells for GFP and the marker. ( f ) High magnification of the rectangle in ( e ). ( h ) Schematic diagram of temporal identity transition of cerebellar GABAergic neuron progenitors from PCPs to PIPs. PCPs at early stages change their character to become PIPs at late embryonic stages and start to generate Pax2+ INs. Scale bars represent: ( a – c , e ) 100 μm, ( f ) 25 μm, ( g ) 10 μm. Full size image One possible explanation for this dynamic change is that, during development, PCPs decrease in number by reduction of the proliferation rate and/or cell death and PIPs increase by enhancement of the proliferation capacity. However, we never detected any apoptotic cells with active caspase 3 in either Olig2+ or Gsx1+ progenitors at E12.5 ( Supplementary Fig. 4a–d ). In addition, we observed no differences in proliferation capacity between Olig2+ and Gsx1+ progenitors at E12.5, as estimated by phosphohistone H3 immunoreactivity ( Supplementary Fig. 4e,f ) and BrdU incorporation rates ( Supplementary Fig. 4g,h ). Therefore, this explanation is not likely. Another explanation for the dynamic change is that PCPs at early neurogenesis stages change their character to become PIPs at later stages. To test this, we performed an ‘Intermediate-term’ lineage trace analysis by using Olig2 GFP/+ embryos. As mentioned above, GFP remains detectable in Olig2-lineage cells for several days, even after the promoter activity of Olig2 gene is downregulated. Therefore, if PCPs at earlier stages give rise to PIPs at later stages, some GFP-labelled cells that lose Olig2 expression might become Gsx1+ cells or Pax2+ INs in Olig2 GFP/+ embryos at later stages. In fact, some GFP-positive cells were found to express Gsx1 at E13.5 ( Fig. 3e,f ) or Pax2 at E14.5 ( Fig. 3g ) in Olig2 GFP/+ cerebellar primordium. Although we could detect many GFP-labelled cells in Pax2-expressing area where postmitotic neurons resided, the number of GFP-labelled cells in the Gsx1-expressing area containing mitotic GABAergic progenitors was not very large. We suspect that residual GFP tended to be diluted by cell division in those mitotic progenitors, or degradation of GFP may occur faster in those cells than in postmitotic neurons. Either way, these results indicate that PCPs change their identity to become PIPs at later stages ( Fig. 3h ). This ‘temporal identity transition from PCPs to PIPs’ seems to gradually take place in a ventral to dorsal direction during development ( Fig. 3d ). It is difficult to determine precisely whether Gsx1 is expressed within the Ptf1a domain at the exact time when Ptf1a starts to be expressed in the cerebellar primordia. However, we did observe that Gsx1 is expressed by a very small population of cells in the ventralmost Ptf1a domain as early as E11.0 and E11.5 ( Supplementary Fig. 5 ). This suggests that, even at the earliest stage of cerebellar GABAergic neuron production, there exist two populations of GABAergic progenitors, PIPs and PCPs, although the number of PIPs is relatively small. PCPs that occupy most of the Ptf1a domain at the earliest stage gradually change their identity to become PIPs at later stages and as a consequence, the Ptf1a domain becomes occupied with PIPs by E14.5. In the rest of the manuscript, we will focus particularly on the temporal identity transition of PCPs to PIPs, although we will also assess the earliest population of PIPs in the Discussion. Investigation of the Gsx1 function in vivo In order to investigate the function of Gsx1 in the temporal identity transition, we generated a mouse line ( pN3-Gsx1 Tg) carrying a transgene that was designed to express Gsx1 under the control of the Neph3 promoter [33] . Because the Neph3 promoter is a direct target of Ptf1a, Gsx1 should be heterochronically expressed in the entire Ptf1a domain even at earlier stages such as E12.5 (ref. 34) [34] . Here, we equally divide the Ptf1a and Lhx1/5+ (c2) domains into three regions along the dorsoventral axis for the sake of convenience: ventral, intermediate and dorsal regions (green, yellow and red lines in Figs 1a–d , 4a–h and 5a,e,i,m ). 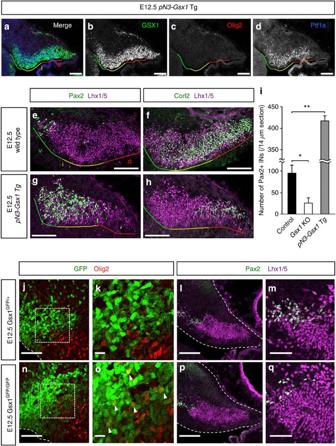Figure 4: Phenotypes ofpN3-Gsx1Tg andGsx1KO mice. (a–d) Cerebellar primordium of E12.5pN3-Gsx1Tg mouse stained with antibodies for Gsx1, Ptf1a and Olig2. Coloured lines indicate ventral (green), intermediate (yellow) and dorsal (red) regions of cerebellar VZ, respectively. (e–h) Cerebellar primordium of E12.5 (e,f) wild-type or (g,h)pN3-Gsx1Tg mouse stained with antibodies for (e,g) Pax2 or (f,h) Corl2 and Lhx1/5. Postmitotic GABAergic neurons are labelled with an antibody for Lhx1/5 at this stage. (i) The average number of Pax2+ INs per slice of control (wild type andGsx1GFP/+),Gsx1GFP/GFPandpN3-Gsx1Tg embryos (n=3, *P<0.05, **P<0.01 byt-test, mean±s.e.m.). (j–q) Immunostaining of E12.5Gsx1GFP/+(j–m) andGsx1GFP/GFP(n–q) cerebella with indicated antibodies. Scale bars represent (a–h,l,p) 100 μm, (j,m,n,q) 50 μm, (k,o) 10 μm. Figure 4: Phenotypes of pN3-Gsx1 Tg and Gsx1 KO mice. ( a – d ) Cerebellar primordium of E12.5 pN3-Gsx1 Tg mouse stained with antibodies for Gsx1, Ptf1a and Olig2. Coloured lines indicate ventral (green), intermediate (yellow) and dorsal (red) regions of cerebellar VZ, respectively. ( e – h ) Cerebellar primordium of E12.5 ( e , f ) wild-type or ( g , h ) pN3-Gsx1 Tg mouse stained with antibodies for ( e , g ) Pax2 or ( f , h ) Corl2 and Lhx1/5. Postmitotic GABAergic neurons are labelled with an antibody for Lhx1/5 at this stage. ( i ) The average number of Pax2+ INs per slice of control (wild type and Gsx1 GFP/+ ), Gsx1 GFP/GFP and pN3-Gsx1 Tg embryos ( n =3, * P <0.05, ** P <0.01 by t -test, mean±s.e.m.). ( j – q ) Immunostaining of E12.5 Gsx1 GFP/+ ( j – m ) and Gsx1 GFP/GFP ( n – q ) cerebella with indicated antibodies. Scale bars represent ( a – h , l , p ) 100 μm, ( j , m , n , q ) 50 μm, ( k , o ) 10 μm. 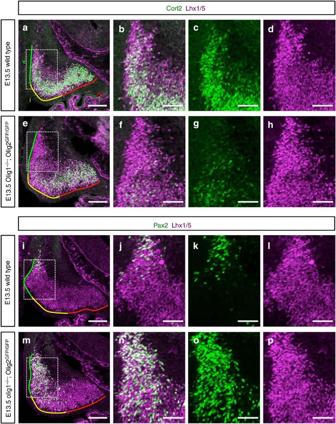Figure 5: Phenotypes ofOlig1/2dKO mice. (a,e) Cerebellar primordium of E13.5 (a) wild-type and (e)Olig1/2dKO mouse stained with antibodies for Corl2 and Lhx1/5. Coloured lines indicate ventral (green), intermediate (yellow) and dorsal (red) regions of cerebellar primordia, respectively. (b–d,f–h) Higher-magnification images of the rectangular regions in (a) and (e), respectively. (i,m) Cerebellar primordium of E13.5 (i) wild-type and (m)Olig1/2dKO mouse stained with antibodies for Pax2 and Lhx1/5. (j–l,n–p) Higher-magnification images of the rectangular regions in (i) and (m), respectively. Scale bars represent (a,e,iandm) 100 μm, (b–d,f–h,j–landn–p) 50 μm. Full size image Figure 5: Phenotypes of Olig1/2 dKO mice. ( a , e ) Cerebellar primordium of E13.5 ( a ) wild-type and ( e ) Olig1/2 dKO mouse stained with antibodies for Corl2 and Lhx1/5. Coloured lines indicate ventral (green), intermediate (yellow) and dorsal (red) regions of cerebellar primordia, respectively. ( b – d , f – h ) Higher-magnification images of the rectangular regions in ( a ) and ( e ), respectively. ( i , m ) Cerebellar primordium of E13.5 ( i ) wild-type and ( m ) Olig1/2 dKO mouse stained with antibodies for Pax2 and Lhx1/5. ( j – l , n – p ) Higher-magnification images of the rectangular regions in ( i ) and ( m ), respectively. Scale bars represent ( a , e , i and m ) 100 μm, ( b – d , f – h , j – l and n – p ) 50 μm. Full size image In these transgenic mice, Gsx1 is expressed by progenitors in the intermediate and dorsal regions of the Ptf1a domain in addition to those in the ventral region at E12.5 ( Fig. 4a–d ). Interestingly, Olig2 expression in the VZ completely disappears in pN3-Gsx1 Tg mice ( Fig. 4c ), indicating that Gsx1 can suppress the expression of Olig2. Next, we examined the effect of induced Gsx1 expression on the differentiation of Pax2+ INs and Purkinje cells. In E12.5 wild-type cerebella, Pax2+ INs reside only in the ventral region of the Lhx1/5+ area (c2 domain, Fig. 4e ). However, in the cerebella of pN3-Gsx1 Tg mice, the distribution of Pax2+ INs is extended to the end of intermediate region of c2 domain at E12.5 ( Fig. 4g ). This indicates that, in addition to progenitors in the ventral region, GABAergic neuron progenitors in the intermediate region also acquired identities of PIPs at this stage in these mice. However, only in rare instances could Pax2+ cells be observed in the dorsal region of the c2 domain, suggesting that PIPs do not reside in the dorsal region of the Ptf1a domain even in the transgenic mice. In E12.5 wild-type cerebella, Corl2+ Purkinje cells were found in the intermediate and dorsal regions of c2 domain but less often in the ventral region ( Fig. 4f ), consistent with the expression pattern of Olig2 at this stage ( Fig. 1d ). In the transgenic mice, Purkinje cells are localized in the dorsal region but less often in the intermediate region and rarely in the ventral region, indicating that PCPs reside in the dorsal region but rarely in the ventral and intermediate regions of the Ptf1a domain ( Fig. 4h ). Together, these findings suggest that PCPs and PIPs reside in the dorsal and intermediate/ventral regions, respectively, in the transgenic mice, while in the wild type, PCPs and PIPs are localized in the dorsal/intermediate and ventral regions of the Ptf1a domain, respectively. To more precisely examine the effect of ectopic Gsx1 expression on the distribution of PCPs and PIPs, we investigated the fate of cerebellar GABAergic neuron progenitors that had undergone final cell division at E11.5. Intraperitoneal injection of BrdU to pregnant dams at E11.5 was performed, and embryos collected at E12.5, followed by immunostaining ( Supplementary Fig. 6a–n ). Statistical analyses revealed that PCPs and PIPs at E11.5 were decreased and increased, respectively, in the pN3-Gsx1 Tg embryos in all cerebellar regions ( Supplementary Fig. 6o,p ). Interestingly, this phenotype is more severe ventrally. Similar results were obtained from transient introduction of Gsx1 into E12.5 cerebella. The Gsx1 and GFP expression vectors were electroporated into the Ptf1a domain at E12.5 and embryos were fixed at E14.5. Among Gsx1-electroporated cells, the ratio of Pax2-expressing cells was increased compared with control ( Supplementary Fig. 7b,d,e ). In contrast, the ratio of Corl2-positive cells was reduced almost to zero ( Supplementary Fig. 7a,c,e ). Because the Gsx1 expression vector contains a strong and ubiquitous promoter [35] , this strong constitutive expression of Gsx1 in progenitors as well as progeny neurons may disturb the normal differentiation into Purkinje cells. Next, we investigated loss–of-function mutants for Gsx1 . In control cerebella ( Gsx1 GFP/+ ) at E12.5, cells that were labelled with Gsx1 promoter-driven GFP never expressed Olig2 ( Fig. 4j,k ). However, many GFP-positive cells at the dorsal edge of the GFP-expressing area were found to express Olig2 in the homozygous cerebella ( Gsx1 GFP/GFP , Fig. 4n,o , arrowheads). This suggests that the cessation of Olig2 expression in GABAergic neuron progenitors was delayed in the absence of Gsx1. Instead, lack of Gsx1 expression might dorsalize these cells leading to prolonged expression of Olig2. Consistently, we also found that Pax2+ INs (Pax2+, Lhx1/5+) were greatly reduced in the Gsx1 GFP/GFP cerebella compared with control heterozygotes ( Fig. 4l,m,p,q ), suggesting a decrease of PIPs in the mutant at this stage. Statistical data on the number of Pax2+ INs in genetic gain- and loss-of-function experiments are shown in Fig. 4i . The proposed function of Gsx1 deduced from the results of these gain- and loss-of-function experiments will be deliberated in the Discussion. Investigation of the Olig2 function in vivo Next we tried to determine the function of Olig2 that is specific for PCPs. First, we examined the phenotype of Olig2 single knockout (KO) mice, but could not detect any abnormalities in the cerebellar primordia except for ectopic expression of Olig1. In the cerebellum of Olig2 KO embryos, Olig1, which was very slightly expressed in the wild-type cerebellum, was upregulated ( Supplementary Fig. 8a–c ). This brought up the possibility that enhanced expression of Olig1 may compensate for Olig2 function in the Olig2 KO mice. Previous reports have indicated that Olig1 could compensate for Olig2 function, at least in some brain regions including midbrain and hindbrain [36] . We therefore investigated the phenotype of Olig1/2 double-KO (dKO) mice ( Supplementary Fig. 8d ). In the E13.5 cerebella of the Olig1/2 dKO mice, we still observed Corl2+ cells ( Fig. 5a,e ). This suggests that Olig2 (and Olig1) are not indispensable for the generation of Purkinje cells. However, the number of Purkinje cells was reduced especially at the ventral and intermediate regions in the dKO cerebellum ( Fig. 5a–h ). Conversely, Pax2+ cells were increased in number, especially at the ventral and intermediate regions ( Fig. 5i–p ). This eventually results in disorganization of the overall structure of the cerebellum as well as Purkinje cell layer at E18.5 in the double mutants ( Supplementary Fig. 8e–j ). To further examine the distribution of PCPs and PIPs in the wild-type and Olig1/2 dKO cerebella at E12.5, we tried to investigate the fate of the cerebellar GABAergic neuron progenitors that had undergone the final cell division at E12.5. Intraperitoneal injection of BrdU to pregnant dams at E12.5 was performed, and embryos collected at E13.5, followed by immunostaining ( Fig. 6a–c ). The distribution and number of BrdU-labelled Purkinje cells and Pax2+ INs were compared between Olig1/2 dKO embryos and control littermates ( Fig. 6d,e ). The ratios of BrdU-labelled Pax2+ INs and BrdU-labelled Corl2+ Purkinje cells to BrdU-labelled Lhx1/5+ cells significantly increased and decreased in Olig1/2 dKO embryos, respectively ( Fig. 6f ). The distribution of BrdU-labelled Pax2+ INs was expanded more dorsally in Olig1/2 dKO embryos. These results indicate that some PCPs in the ventral and intermediate regions are converted to PIPs at E12.5 in the absence of Olig1/2 expression. Indeed, we observed that the ventral portion of cells expressing Olig2 promoter-driven GFP became Pax2+ INs in Olig1/2 dKO embryos at E12.5 ( Fig. 6h ), which was never observed in the heterozygous mice ( Fig. 6g ). 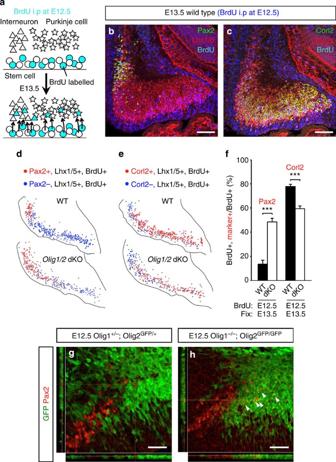Figure 6: Altered fates of GABAergic neurons generated around E12.5 in Olig1/2 dKO mice. (a) Schematic diagram of BrdU incorporation experiment. At E12.5, intraperitoneal injection of BrdU was performed and cells in S-phase (progenitors) incorporated BrdU. At E13.5 postmitotic neurons generated from BrdU-labelled progenitors can also be labelled with BrdU. The number and the position of BrdU-labelled GABAergic interneurons and Purkinje cells predicts a general distribution of PIPs and PCPs at E12.5, respectively. (b,c) Examples of immunostaining of E13.5 wild-type cerebellum using antibodies for BrdU, Lhx1/5 and (b) Pax2 or (c) Corl2. Immunostaining of Lhx1/5 enables the distinction of BrdU-labelled postmitotic neurons from BrdU-labelled mitotic progenitors. (d,e) Representative images of plots of indicated cells in wild-type andOlig1/2dKO cerebella. (f) The ratio of BrdU-labelled Pax2+ INs or Purkinje cells to BrdU-labelled GABAergic neurons in wild-type andOlig1/2dKO cerebella (n=3, ***P<0.001 byt-test, mean±s.e.m.). (g,h) Short-term lineage tracing analyses using (g) heterozygotes and (h) homozygotes ofOlig1/2dKO line. Arrowheads indicate GFP-positive Pax2 INs. Scale bars represent (b,c) 100 μm, (g,h) 25 μm. Figure 6: Altered fates of GABAergic neurons generated around E12.5 in Olig1/2 dKO mice. ( a ) Schematic diagram of BrdU incorporation experiment. At E12.5, intraperitoneal injection of BrdU was performed and cells in S-phase (progenitors) incorporated BrdU. At E13.5 postmitotic neurons generated from BrdU-labelled progenitors can also be labelled with BrdU. The number and the position of BrdU-labelled GABAergic interneurons and Purkinje cells predicts a general distribution of PIPs and PCPs at E12.5, respectively. ( b , c ) Examples of immunostaining of E13.5 wild-type cerebellum using antibodies for BrdU, Lhx1/5 and ( b ) Pax2 or ( c ) Corl2. Immunostaining of Lhx1/5 enables the distinction of BrdU-labelled postmitotic neurons from BrdU-labelled mitotic progenitors. ( d , e ) Representative images of plots of indicated cells in wild-type and Olig1/2 dKO cerebella. ( f ) The ratio of BrdU-labelled Pax2+ INs or Purkinje cells to BrdU-labelled GABAergic neurons in wild-type and Olig1/2 dKO cerebella ( n =3, *** P <0.001 by t -test, mean±s.e.m.). ( g , h ) Short-term lineage tracing analyses using ( g ) heterozygotes and ( h ) homozygotes of Olig1/2 dKO line. Arrowheads indicate GFP-positive Pax2 INs. Scale bars represent ( b , c ) 100 μm, ( g , h ) 25 μm. Full size image We further investigated the distribution of PCPs and PIPs at other developmental stages (E11.5 or E13.5), by performing basically identical experiments where BrdU was administered at E11.5 or E13.5 and embryos were analysed one day later ( Supplementary Fig. 9a–d ). Compared with embryos treated with BrdU at E12.5, similar trends were observed in E11.5 and E13.5 BrdU-administered embryos. The ratios of BrdU-labelled Pax2+ INs and BrdU-labelled Corl2+ Purkinje cells to BrdU-labelled Lhx1/5+ cells significantly increased and decreased in Olig1/2 dKO embryos, respectively, regardless of the date of BrdU administration ( Supplementary Fig. 9e,f ). On the other hand, the production of total cerebellar GABAergic neurons was similar regardless of the date of BrdU incorporation ( Supplementary Fig. 9g ). These findings demonstrate that the decrease and increase of PCPs and PIPs, respectively, during cerebellar development was accelerated in the Olig1/2 dKO mice and therefore suggest that temporal identity transition from PCPs to PIPs was accelerated in the mutants. Overall, these results lead to the notion that Olig2 may act as a brake for temporal identity transition ( Fig. 7i ). 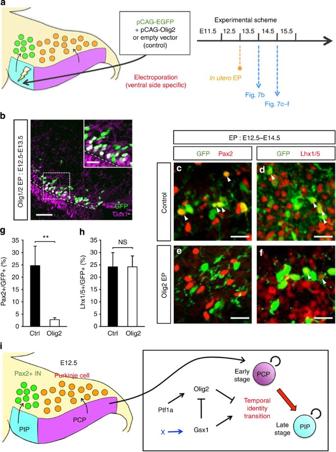Figure 7: Ectopic expression of Olig2 in Gsx1-expressing progenitors. (a) Schematic diagram ofin uteroelectroporation. Plasmid DNA was injected into the fourth ventricle and electroporated to the Gsx1-expression region at E12.5. The electroporated brains were collected at E13.5 or E14.5. (b) Immunostaining of E13.5 wild-type cerebellum electroporated with Olig2 at E12.5. Antibodies are indicated. (c–f) Sections of E14.5 wild-type mice electroporated with (c,d) control and (e,f) Olig2. Regions just above the Gsx1-expressing cells are shown. Arrowheads indicate co-immunostaining of GFP and the marker. (g,h) Quantification of the percentages of (g) Pax2-positive cells and (h) Lhx1/5-positive cells in electroporated cells (n=3, NS, not significant, **P<0.01 byt-test, mean±s.e.m.). (i) Summary of this study. Scale bars represent (b) 25 μm, (inset ofb,c–f) 10 μm. Figure 7: Ectopic expression of Olig2 in Gsx1-expressing progenitors. ( a ) Schematic diagram of in utero electroporation. Plasmid DNA was injected into the fourth ventricle and electroporated to the Gsx1-expression region at E12.5. The electroporated brains were collected at E13.5 or E14.5. ( b ) Immunostaining of E13.5 wild-type cerebellum electroporated with Olig2 at E12.5. Antibodies are indicated. ( c – f ) Sections of E14.5 wild-type mice electroporated with ( c , d ) control and ( e , f ) Olig2. Regions just above the Gsx1-expressing cells are shown. Arrowheads indicate co-immunostaining of GFP and the marker. ( g , h ) Quantification of the percentages of ( g ) Pax2-positive cells and ( h ) Lhx1/5-positive cells in electroporated cells ( n =3, NS, not significant, ** P <0.01 by t -test, mean±s.e.m.). ( i ) Summary of this study. Scale bars represent ( b ) 25 μm, (inset of b , c – f ) 10 μm. Full size image Interestingly, pN3-Gsx1 Tg and Olig1/2 dKO embryos exhibit similar phenotypes; decrease and increase of PCPs to PIPs, respectively. We compared the total number of Corl2- or Pax2-expressing cells between the E12.5 cerebella of pN3-Gsx1 Tg and Olig1/2 dKO embryos that were administered with BrdU at E11.5. Statistical analysis clearly showed that the phenotype is much more severe in pN3-Gsx1 Tg embryos than Olig1/2 dKO mice ( Supplementary Fig. 9h ). Next, we examined whether ectopic expression of Olig2 in PIPs suppresses the expression of Gsx1. Olig2 expression vector was co-electroporated with the GFP expression vector into the ventral region of the Ptf1a domain at E12.5, and brains were harvested at E13.5 ( Fig. 7a ). We found that ectopically expressed Olig2 could not suppress the expression of Gsx1 in the ventral region ( Fig. 7b ), although Gsx1 can suppress the expression of Olig2 when ectopically expressed ( Fig. 4a–d ). In those cells electroporated with the Olig2 vector, both Olig2 and Gsx1 were expressed simultaneously ( Fig. 7b ). We examined the types of neurons that were generated from progenitors expressing both transcription factors. Two days after the electroporation at E12.5, brains were collected for immunostaining ( Fig. 7a ). In the control brains, some of electroporated cells expressed the interneuron marker Pax2 ( Fig. 7c,g ). However, when co-electroporated with the Olig2 expression vector, Pax2 expression was rarely observed ( Fig. 7e,g ). On the other hand, the expression of Lhx1/5, a marker for all cerebellar GABAergic neurons, was similar between control and Olig2-overexpressed brains ( Fig. 7d,f,h ). These results indicate that forced expression of Olig2 in PIPs inhibits proper differentiation to Pax2+ INs. Previous studies showed that high expression of Olig2 blocks neuronal maturation [37] , therefore it is likely the strong ectopic promoter-driven Olig2 expression in this experiment inhibits proper differentiation of Pax2+ INs. Genetic interaction of Olig2, Gsx1 and Ptf1a expression Finally, we examined genetic interaction between Olig2, Gsx1 and Ptf1a. Ptf1a is known as an indispensable transcription factor for GABAergic neuron specification in the cerebellum [7] . The expression of Olig2 disappeared specifically in the VZ of Ptf1a KO embryos, although its expression at the pial side was not affected ( Supplementary Fig. 10a–f ), suggesting that Olig2 may be a downstream target of Ptf1a in the VZ ( Fig. 7i ). Next, we utilized another null allele for the Ptf1a gene ( Ptf1a YFP ) in which the Ptf1a domain is labelled by a Ptf1a promoter-driven YFP. In contrast to Olig2 expression, the expression of Gsx1 was maintained in the YFP-positive area of Ptf1a -null embryos ( Ptf1a YFP/YFP ) ( Supplementary Fig. 10g–r ), suggesting that there may be another upstream regulator for Gsx1 ( Fig. 7i ). In the Ptf1a -null cerebella ( Ptf1a YFP/YFP ) at E13.5, we could not detect any GABAergic inhibitory neurons that were labelled with the specific marker, Lhx1/5 ( Supplementary Fig. 10s,t ), consistent with previous findings that no GABAergic neurons were produced in the Ptf1a mutants [5] . Accordingly, in the Ptf1a -mutant cerebella ( Ptf1a YFP/YFP ), Pax2+ INs were not observed in the Ptf1a lineage, which were labelled with GFP ( Supplementary Fig. 10s,t ). In this study, we found there are two distinct subpopulations in cerebellar GABAergic neuron progenitors within the Ptf1a domain at E12.5; dorsally located Olig2+ and ventrally localized Gsx1+ progenitors. Short-term lineage analyses with GFP-knock-in mice revealed that Olig2+ and Gsx1+ progenitors are PCPs and PIPs, respectively. Furthermore, our intermediate lineage trace analysis using Olig2 GFP/+ mice showed that PCPs at earlier stages change their character to become PIPs at later stages. We termed this change as ‘temporal identity transition’ of cerebellar GABAergic progenitors. Furthermore, it seems that temporal identity transition occurs earlier ventrally and later dorsally, because Gsx1-positive cells first appear in the ventral side and later in the dorsal side of the Ptf1a domain at corresponding developmental stages. However, our data also implied that a small number of cells express Gsx1 at the most ventral region of the Ptf1a domain at a very early stage, while many more cells express Olig2 within the Ptf1a domain. Because a previous study reported that Pax2+ INs in the DCN can be produced as early as Purkinje cells [14] , these ventrally located Gsx1+ cells may be PIPs that produce Pax2+ INs in the DCN. Therefore, one might imagine that there are two distinct spatially defined regions within the Ptf1a domain at the onset of GABAergic neuron production; a small number of PIPs at the ventral most region and large number of PCPs in the other regions of the Ptf1a domain. As development proceeds, those PCPs gradually change their identity to become PIPs from ventral to dorsal, until the entire Ptf1a domain is occupied with PIPs by E14.5. Because we were interested in the temporal identity transition from PCPs to PIPs, we focused on that issue in this study. Muguruma et al. [38] previously succeeded in differentiating ES cells into cerebellar GABAergic neurons. During culture after certain induction procedures, Corl2+ cells are first produced and subsequently Pax2+ cells are generated in cells derived from an ES cell clone. Although that experiment did not directly show that ES-derived PCPs and PIPs are in the same lineage, ES cell-derived PCPs likely also change into PIPs during culturing, given our in vivo findings in this study. After the initial induction steps, no extrinsic factors appear to be required to elicit the temporal identity change in vitro . This suggests that cerebellar GABAergic progenitors have their own internal clocks that carry temporal information to elicit the temporal identity transition at the appropriate time. Because the temporal identity transition from PCPs to PIPs occurs earlier at the ventral side, the internal clocks of cerebellar GABAergic progenitors may be faster in the ventral region and slower in the dorsal region. We observed that some Purkinje cells were produced in the Olig1/2 dKO mice, suggesting that Olig2 (and Olig1) might not be indispensable for Purkinje cell generation. However, Purkinje cells and Pax2+ INs were decreased and increased, respectively, especially at the ventral and intermediate regions. Moreover, BrdU incorporation studies at different developmental stages showed that both the decrease and increase of PCPs and PIPs, respectively, during cerebellar development were accelerated in the mutant mice. These findings suggest that temporal identity transition from PCPs to PIPs was accelerated in the mutants and therefore suggest that Olig2 (and Olig1) may function as a brake for the temporal identity transition as well as the internal clocks of GABAergic neuron progenitors. The milder phenotype at the dorsal side could be explained from the viewpoint of internal clocks as follows. The internal clocks of dorsally located progenitors are set later than those of ventrally or intermediately localized progenitors in the wild-type mice, acceleration of the internal clocks by loss of Olig2 (and Olig1) may not be sufficient to elicit the temporal identity transition in the dorsal region. In neither Olig2 GFP/+ nor Olig1 +/− ; Olig2 GFP/+ cerebella at E12.5, did we ever observe Pax2+ INs that were labelled with GFP. This may imply that the temporal identity transition from PCPs to PIPs do not occur prior to the stage that these Pax2+ INs are produced (for example, E11.5). However, in Olig1/2 dKO cerebella at E12.5, we observed many GFP-labelled Pax2+ INs. This finding also suggests that the temporal identity transition precociously occurs in the dKO mice. A gain–of-function experiment using BrdU-injected pN3-Gsx1 Tg mice showed that forced expression of Gsx1 caused a decrease and increase of PCPs and PIPs, respectively, at an early stage (E11.5). This phenotype was more severe at the ventral/intermediate regions but milder in the dorsal region. Two explanations are possible for this phenotype. One is that Gsx1 gives ventralizing spatial information to GABAergic neuron progenitors and gain of this function leads to ventralization of the GABAergic progenitors causing their ectopic transition to PIPs. The other explanation is that Gsx1 may act as an accelerator for the temporal identity transition as well as the internal clocks of GABAergic neuron progenitors and gain of this function results in precocious temporal identity transition from PCPs to PIPs. We also observed many Olig2-expressing cells within the GFP-labelled region in Gsx1 GFP/GFP embryonic cerebella, which are never found in control Gsx1 GFP/+ . Consistently, the number of Pax2+ INs was remarkably reduced in the homozygous mutants at E12.5. Similar to the results from the pN3-Gsx1 Tg mice, this phenotype can also be likewise interpreted. Gsx1 may give ventralizing information to GABAergic progenitors and loss of this function leads to dorsalization of GABAergic progenitors inhibiting their transition to PIPs. Or, Gsx1 may act as an accelerator for the internal clocks and loss of this function results in delayed temporal identity transition. Actually, it is difficult to discriminate between these two possibilities. However, because Olig2 and Gsx1 are expressed in a complementary pattern and because the loss–of-function mutants for the two genes exhibit opposite phenotypes, it is likely that Olig2 and Gsx1 have opposing functions. As Olig2 was revealed to function as a brake for the temporal identity transition, we predict that Gsx1 may function as an accelerator for it. However, further investigation is required. This study showed that Gsx1 suppresses the expression of Olig2, but that Olig2 cannot suppress Gsx1 expression. This raises a possibility that the accelerating effect on temporal identity transition by Gsx1 may be accomplished through downregulation of Olig2 expression, because Olig2 works as a brake for temporal identity transition. However, we believe Gsx1 may not only suppress the expression of Olig2 but it may work via some additional pathways for the progression of temporal identity transition, because the severity was much greater in pN3-Gsx1 Tg than in Olig1/2 dKO mice ( Supplementary Fig. 9h ). In addition, forced expression of Olig2 in PIPs using an expression vector with a strong promoter cannot suppress the expression of Gsx1. Actually, few cells were observed to express both proteins in the Ptf1a domain. Therefore, the asymmetry in genetic interaction between the expression of Olig2 and Gsx1 may enable the unidirectional progression of temporal identity transition from the ventral region to the dorsal region. In addition, we showed that Ptf1a is required for the expression of Olig2 but not for that of Gsx1. The genetic relationship among transcription factors is summarized in Fig. 7i . In vertebrates and invertebrates, it is likely that neuronal progenitors have two types of identities; spatial and temporal. In fruitflies, one hemineuromere has about 30 neuroblasts, which are localized in spatially distinct locations, express different sets of transcription factors and produce distinct types of neurons and glia [39] , [40] . Moreover, each neuroblast changes its temporal identity during development, to generate various neurons/glia types [41] . Many studies have been done to investigate the temporal identities of neuroblasts in Drosophila , revealing the involvement of transcription factors such as Hunchback, Krüppel, Pdm and Castor in defining the temporal identities of neuroblasts. In addition to such ‘temporal identity determinants’, several ‘temporal identity transition regulators’ like Seven up, Dan/Danr, and so on, which control the speed of progression of temporal identity transition have been identified [42] . In the mammalian telencephalon, glutamatergic and GABAergic neurons are generated from spatially distinct progenitors; dorsal and ventral neuroepithelia, respectively [43] . Their spatial identities are thought to be defined by bHLH transcription factors, such as Neurogenin1/2 and achaete-scute complex-like 1 (also called Mash1). In addition, even from the same neuroepithelial regions in the dorsal telencephalon, different types of neurons can be produced; early-born and late-born neurons differentiate into deep-layer and superficial-layer neurons, respectively, with distinct characteristics [44] . This indicates that the temporal identity of glutamatergic progenitors varies as development proceeds. However, the molecular mechanisms controlling the temporal identities in mammals are still elusive. In the mammalian cerebellar primordium, we and others have previously suggested that two bHLH proteins, Atoh1 and Ptf1a are involved in specifying the spatial identities of neural progenitors [5] , [6] , [7] , [45] . In this work, we found two types of GABAergic progenitors, PCPs and PIPs, which are in the same lineage but have distinct temporal identities. Unfortunately, the temporal identity determinants for PCPs and PIPs remain elusive, as the presence of Purkinje cells or Pax2+ INs in either loss of Olig2 or Gsx1 gene could still be observed. However, we believe that we have found candidates for the temporal identity transition regulators that negatively and positively control the speed of the temporal identity transition of GABAergic neuron progenitors. There are thousands of neuron types in the nervous system, each of which has morphologically, electrophysiologically and immunohistochemically distinct characteristics. Although the diversity of neurons may be, at least in part, explained by the diversity of spatial and temporal identities of neuronal progenitors, the underlying molecular machinery is still elusive, especially regarding the temporal identities in vertebrates. Further studies are required to understand the molecular mechanisms that produce the variety of neuronal types. Animals All animal experiments in this study have been approved by the Animal Care and Use Committee of the National Institute of Neuroscience, Japan. Ptf1a YFP , Ptf1a Cre lines were described previously [46] , [47] , [48] . Olig2 GFP and Gsx1 GFP lines were generated by replacing the ORF sequence of each gene with GFP cDNA, respectively. Olig1 null Olig2 GFP was generated by deleting the ORF of Olig1 gene and replacing the ORF sequence of Olig2 gene with GFP cDNA (see also Supplementary Figs 2,5 ). pN3-Gsx1 Tg was generated by a standard method [49] . A quantity of 3.5 ng μl −1 of linearized and agarose gel purified plasmid DNA was microinjected into pronuclei of fertilized eggs derived from the superovulated B6C3F1 mouse strain (SLC, Japan). The construct for this line was generated by inserting the ORF sequence of Gsx1 into a pN3 vector. Antibodies and immunohistochemistry Primary antibodies used in this study were anti-BrdU (1:200; rat; ABD Serotec, Kidlington, UK), Corl2 (1:500; rabbit polyclonal), GFP (1:10; rat; a kind gift from Dr A. Imura, Kyoto University, Kyoto, Japan), Gsx1 (1:250; rat), Lhx1/5 (1:3,000; mouse; DSHB, Iowa City, IO, USA), Olig2 (1:500; goat; R&D Systems, Minneapolis, MN, USA), Pax2 (1:200; rabbit; Invitrogen, Carlsbad, CA, USA), Ptf1a (1:200; rabbit), RORa (1:2,000; goat; Santa Cruz Biotechnology, Santa Cruz, CA, USA). Rat monoclonal anti-Gsx1 mAb was raised against GST-Gsx1 1-72 amino acids (aa). Anti-Ptf1a antibody was generated as follows. The fragment of mouse Ptf1a full length (Full: 1–324 aa) or -amino-terminal (NT: 1–145 aa) was inserted into pMAL-c2 (New England Laboratories, Beverly, MA) or pGEX-4T-2 (Amersham Pharmacia Biotech, Buckinghamshire, UK), respectively. Maltose-binding protein and glutathione S -transferase (GST) fusion proteins were expressed in Escherichia coli BL21 (DE3) and purified according to the manufacturer’s instructions. Polyclonal rabbit anti-Ptf1a antibody was prepared against maltose-binding protein-Ptf1a-Full as an antigen, and then purified by use of GST-Ptf1a-NT. This antibody detected no signals in the Ptf1a -null ( Ptf1a Cre/Cre ) mutant. Immunohistochemistry was performed as follows. Embryos were fixed with 4% paraformaldehyde in PBS. After the cryoprotection, embryos were embedded in OCT compound. Cryosections were made in the thickness of 14 μm. Sections were treated with 0.5% BSA in PBS containing 0.2% Triton X-100 (blocking buffer) at room temperature for 1 h and subsequently incubated with antibodies listed below in blocking buffer at 4 °C for 20 h. Specimens were subsequently rinsed with PBS and incubated with the secondary antibody at room temperature for 2 h. Tissues were examined by fluorescent microscopy. Coloured lines that divide VZ or c2 domain (where cerebellar GABAergic neurons reside) into ventral (green), intermediate (yellow) and dorsal (red) in Figs 1 , 4 , 5 , were drawn by equally dividing the length of the bottom of VZ or c2 domain by three. Dashed lines that divide c2 domain into ventral, intermediate and dorsal area in Supplementary Fig. 6 were drawn perpendicularly to the tangent of the points, which equally divide the length of the bottom of c2 domain by three. BrdU incorporation experiment Pregnant mice (E11.5, E12.5 and E13.5) were given intraperitoneal injections of BrdU at 100 mg kg −1 . Twenty-four hours after the BrdU injection, embryos were fixed and subjected to immunohistochemical analyses as follows. After the immunostaining with antibodies besides BrdU, sections were post-fixed with 4% paraformaldehyde in PBS at room temperature for 20 min. After the fixation, sections were treated with 2N hydrochloric acid at 37 °C for 30 min. Then sections were washed and immunostaining with anti-BrdU was performed. The number of BrdU, Lhx1/5-double-positive cells and BrdU, Lhx1/5, Corl2 (or Pax2)-triple-positive cells were quantified. BrdU, Lhx1/5-double-positive cells were counted as neurons generated during the 24 h after the BrdU injection. By calculating the rate of triple-positive cells to double-positive cells and plotting the positions of these cells, we roughly estimated the number and distribution of PCPs and PIPs in the progenitor domain at the injected stages. To analyse the BrdU incorporation rates of PIPs and PCPs in E12.5 wild-type embryos, pregnant mice (E12.5) were given two intraperitoneal injections of BrdU at 50 mg kg −1 with a 30-min interval. One hour after the first BrdU injection, mice were killed and embryonic brains were fixed and subjected to immunohistochemical analyses. In utero electroporation One microliter of plasmid DNA (mixture of pCAG-EGFP-N3: 0.5 mg ml −1 and pCAG-Olig2: 1 mg ml −1 or pCAG-Gsx1: 1 mg ml −1 ) in TE (Tris-EDTA; 10 mM Tris, 1 mM EDTA, pH 7.5) containing Fast Green was injected into the fourth ventricles of embryonic brains from outside the uterus with a glass micropipette (G-1.0; Narishige). Holding the embryo in utero with forceps-type electrodes (NEPA GENE), 50 ms of 40 V electronic pulses were delivered five times at intervals of 450 ms with a square electroporator (Nepa Gene). pCAG-Olig2 and pCAG-Gsx1 vector was generated by inserting the ORF sequence into the cloning site of pCAG2-en. How to cite this article : Seto, Y. et al. Temporal identity transition from Purkinje cell progenitors to GABAergic interneuron progenitors in the cerebellum. Nat. Commun. 5:3337 doi: 10.1038/ncomms4337 (2014).